Mid-infrared optical frequency combs at 2.5 μm based on crystalline microresonators The mid-infrared spectral range ( λ ~2–20 μm) is of particular importance as many molecules exhibit strong vibrational fingerprints in this region. Optical frequency combs—broadband optical sources consisting of equally spaced and mutually coherent sharp lines—are creating new opportunities for advanced spectroscopy. Here we demonstrate a novel approach to create mid-infrared optical frequency combs via four-wave mixing in a continuous-wave pumped ultra-high Q crystalline microresonator made of magnesium fluoride. Careful choice of the resonator material and design made it possible to generate a broadband, low-phase noise Kerr comb at λ =2.5 μm spanning 200 nm (≈10 THz) with a line spacing of 100 GHz. With its distinguishing features of compactness, efficient conversion, large mode spacing and high power per comb line, this novel frequency comb source holds promise for new approaches to molecular spectroscopy and is suitable to be extended further into the mid-infrared. Optical frequency combs [1] , [2] , that is, broad spectral bandwidth coherent light sources consisting of equally spaced sharp lines, revolutionized optical frequency metrology one decade ago. They now enable dramatically improved acquisition rates, resolution and sensitivity for molecular spectroscopy mostly in the visible and near-infrared ranges [3] , [4] , [5] , [6] , [7] , [8] . The mid-infrared spectral range ( λ ~2–20 μm) is known as the ‘molecular fingerprint’ region as many molecules have their characteristic, fundamental vibrational bands in this part of the electromagnetic spectrum. Broadband mid-infrared spectroscopy therefore constitutes a powerful and ubiquitous tool for optical analysis of chemical components that is used in biochemistry, astronomy, pharmaceutical monitoring and material science. Mid-infrared frequency combs have therefore become highly desirable and recent progress in generating such combs by nonlinear frequency conversion [9] , [10] , [11] has opened access to this spectral region. Because of its scientific and technological significance, laser technology in the mid-infrared is an active area of research and development. The advent of a compact and versatile coherent light source in this region came after the invention of quantum cascade lasers (QCLs) in 1994 (ref. 12 ). However, QCLs are intrinsically difficult to be passively mode-locked [13] and only active mode-locking has been unequivocally demonstrated, creating a limited comb-like spectrum of ~0.3 THz bandwidth [14] . Today, the most common approach to create frequency combs in the mid-infrared is to frequency down-convert a near-infrared comb through nonlinear processes, such as optical parametric oscillation [9] , [10] or difference frequency generation [11] . In this article, we demonstrate a novel, direct route to mid-infrared frequency comb generation based on ultra-high Q (quality factor) crystalline optical microresonators [15] . The particular advantages of microresonator-based frequency combs are the compact form factor, large comb mode spacing and high power per comb line. The underlying mechanism is cascaded four-wave mixing caused by the third-order Kerr nonlinearity in high-Q whispering-gallery mode (WGM) microresonators, which was first demonstrated in silica microtoroids in the near infrared [16] , [17] . In this energy-conserving process, two possibly degenerate photons (frequency ν 1 and ν 2 ) are converted to a pair of signal ( ν S ) and idler ( ν I ) photons, such that ν 1 + ν 2 = ν S + ν I . This process can cascade and thereby lead to the formation of an equidistant optical frequency comb (‘Kerr’ comb), whose spectral properties (offset frequency and mode spacing) can be stabilized [18] . Several microresonator platforms based on this mechanism have demonstrated Kerr frequency comb generation in the near-infrared region [15] , such as silica microtoroids [17] , [18] , [19] , silicon nitride [20] , [21] , Hydex glass [22] , crystalline fluorides [23] , [24] and fused quartz [25] , where most optical materials are transparent and characterized by close-to-zero anomalous dispersion. Most of the platforms, however, principally cannot operate in the mid-infrared region. Here, by careful choice of resonator material and design, we demonstrate for the first time mid-infrared Kerr frequency combs based on microresonators. In addition, we have carefully characterized their phase noise and shown that the mid-infrared Kerr combs indeed consist of narrow and mutually coherent lines. The current approach is suitable for extending comb generation further into the mid-infrared. Crystalline Resonator fabrication and characterization We developed ultra-high Q resonators made of crystalline magnesium fluoride MgF 2 for mid-infrared frequency comb generation. The reason for choosing MgF 2 is threefold. First, the transparency window of crystalline materials (such as CaF 2 and MgF 2 ) extends from the ultraviolet (~160 nm) to the mid-infrared (~7 μm), enabling achievement of ultra-high Q (>10 8 ) optical modes in the mid-infrared—in contrast to fused silica or quartz, which exhibit strong absorption above 2.2 μm. Second, the ability to generate optical frequency combs via cascaded four-wave mixing in the presence of self- and cross-phase modulation of the pump requires the group velocity dispersion (GVD) at the pump frequency to be anomalous [16] , [26] , [27] , that is, a free spectral range (FSR) of the cavity that reduces with increasing wavelength. We assess the dispersion properties by carrying out fully vectorial finite element simulations [28] , [29] taking into account geometric effects as well as the intrinsic material dispersion. The resonator dispersion is expressed via the parameter D 2 =2 π ( ν m +1 −2 ν m + ν m −1 ), where ν m is the resonance frequency with azimuthal mode number m . 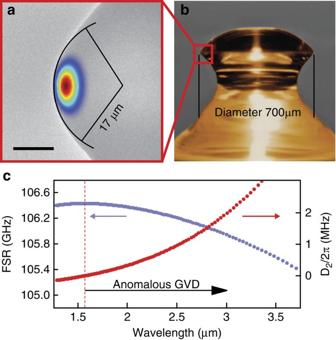Figure 1: Properties of a MgF2crystalline WGM microresonator. (a) Finite element simulation of the optical intensity profile of the fundamental WGM at wavelength 2.45 μm superimposed on a scanning electron microscope image of a 700-μm diameter resonator used in this work, fabricated by polishing and shaping an ultraviolet-grade MgF2cylinder blank. Scale bar, 10 μm. The radius of curvature of the resonator protrusion, which confines the WGM in the azimuthal direction, is 17 μm. (b) Optical microscope image of the resonator. (c) The figure shows the simulated FSR for fundamental modes with mode numberm(FSRm=(νm+1−νm−1)/2, blue curve) and the difference of the FSR between adjacent modes (D2/2π=νm+1−2νm+νm−1, red curve) as a function of the wavelength for the resonator in panela, exhibiting an anomalous GVD (D2>0) aboveλ=1.6 μm. Figure 1b shows a 700-μm-diameter MgF 2 crystalline resonator with its dispersion properties shown in Fig. 1c , revealing a GVD that is anomalous over the full mid-infrared transparency range. In contrast to previous work in crystalline (and other) resonators, the present experiments operate in the strongly anomalous dispersion region ( D 2 ~ κ , where κ is the cavity decay rate). We emphasize that this dispersion region—far from the zero dispersion point, which is at about 1.55 μm—has previously been considered as unfavourable for Kerr comb generation [17] , [20] , [23] due to the mismatch between cavity resonances and equidistant comb lines. Here, we experimentally demonstrate that the strong anomalous dispersion does not prevent broadband Kerr comb generation in the mid-infrared region. This can be attributed to the nonlinear frequency pulling by self- and cross-phase modulation exceeding the amount of cavity dispersion. Moreover, as detailed below and recently reported [30] , sufficiently high anomalous dispersion is one way to achieving low-phase noise operation of the comb. The requirement for anomalous dispersion renders other materials, such as Si 3 N 4 microring resonators, which are used successfully at shorter wavelength for Kerr comb generation, unfavourable as their GVD is normal in the mid-infrared [31] . Third, the sign of the temperature coefficient of the refractive index (d n /d T ) and the thermal expansion coefficient α are both positive in MgF 2 (at room temperature), which allows the cavity mode to be thermally self-locked to the pump laser frequency [32] and enables the stabilization of the repetition rate and offset frequency of microresonator-based frequency combs [18] . On the contrary, materials with opposite signs of d n /d T and α , such as CaF 2 , suffer from large thermal oscillatory instabilities and the requirement for active locking (or injection locking) schemes (see Supplementary Note for more information on thermal instability). Figure 1: Properties of a MgF 2 crystalline WGM microresonator. ( a ) Finite element simulation of the optical intensity profile of the fundamental WGM at wavelength 2.45 μm superimposed on a scanning electron microscope image of a 700-μm diameter resonator used in this work, fabricated by polishing and shaping an ultraviolet-grade MgF 2 cylinder blank. Scale bar, 10 μm. The radius of curvature of the resonator protrusion, which confines the WGM in the azimuthal direction, is 17 μm. ( b ) Optical microscope image of the resonator. ( c ) The figure shows the simulated FSR for fundamental modes with mode number m (FSR m =( ν m +1 − ν m −1 )/2, blue curve) and the difference of the FSR between adjacent modes ( D 2 /2 π = ν m +1 −2 ν m + ν m −1 , red curve) as a function of the wavelength for the resonator in panel a , exhibiting an anomalous GVD ( D 2 >0) above λ =1.6 μm. Full size image To fabricate the resonators, single-crystal ultraviolet-grade MgF 2 was first cut into cylinder blanks with dimensions of several millimetres. The resonators were then shaped and polished on an air-bearing spindle by diamond abrasives to achieve a smooth protrusion which provides an azimuthal WGM confinement, following the methods described in detail in ref. 33 . A scanning electron microscope was used to measure the transverse radius of curvature of the resonator of 17 μm ( Fig. 1a ). The resulting mode area of the WGM was determined in a fully vectorial finite element simulation. Superimposed on Fig. 1a is the intensity profile of the fundamental mode at λ =2.45 μm. From these simulations, we obtained an effective mode area A eff =60 μm 2 and determined the effective nonlinearity of the resonator γ eff =2π n 2 /( λ A eff )=4.3 × 10 −4 m −1 W −1 , where n 2 is the Kerr nonlinearity of MgF 2 (1 × 10 −20 m 2 W −1 ). The diameters of the resonators typically range from 500 μm to 5 mm, corresponding to a resonator mode spacing in the range of 10–110 GHz. Tapered optical fibres made of silica were used for characterization of the resonators at 1.55 μm. For pre-characterization, the quality factor of the resonances was measured with a tuneable, narrow-linewidth (short-term<100 kHz) fibre laser at λ =1.55 μm, yielding intrinsic Q factors exceeding 10 9 , corresponding to a typical finesse of F =10 5 –10 6 . Additional iterative thermal annealing and polishing steps may further increase the Q factors [34] . Generation of mid-infrared frequency comb We pumped the resonators by a continuous-wave (CW) mid-infrared laser based on an optical parametric oscillator that is tuneable between 2.4 and 2.5 μm with short-term linewidth<100 kHz. Details of the laser source and the experimental set-up can be found in the Methods section and in Fig. 2a . Optical power levels of 200 mW to 1 W were coupled into the resonators by employing a tapered fibre made of low-OH-fused silica (loss ~3.4 dB m −1 at λ =2.5 μm). The resonator and tapered fibre are embedded in a dry-nitrogen-purged environment, as water vapour is highly absorptive in the mid-infrared (prior exposure to air however is not expected to lead to accumulation of water layers as MgF 2 crystals are hydrophobic). The output spectra were recorded by an optical spectrum analyser (OSA) with cut-off wavelength at 2.5 μm. 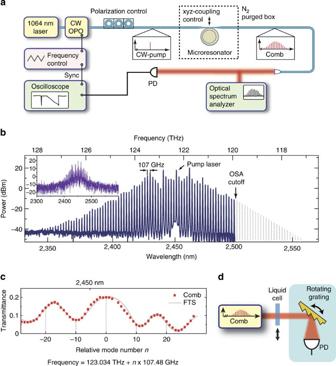Figure 2: Mid-infrared optical frequency comb generation using a crystalline MgF2microresonator. (a) The experimental set-up consists of a CW mid- infrared OPO that serves as the pump laser. The pump laser is coupled via a tapered fibre to a crystalline MgF2microresonator. The generated frequency comb is detected using an optical spectrum analyser (OSA) with a cut-off wavelength of 2.5 μm (PD, photodetector). (b) Frequency comb spectrum recorded by the OSA aroundλ=2.45 μm with a line spacing of 107 GHz generated from pumping a 700-μm-diameter MgF2resonator (pump power 600 mW). The grey lines denote frequency components, which are expected to exist based on symmetry around the pump. Inset shows the spectrum taken with a Fourier transform spectrometer, which reveals the overall symmetry of the spectrum. (c) Proof-of-principle mid-infrared Kerr comb absorption spectroscopy experiment. The figure shows the transmittance of 0.5-mm-thick liquid acetone (single-pass) recorded as the relative intensities of the attenuated and unattenuated Kerr comb (shown in panelb) line intensities (red dot) and independently by a Fourier transform spectrometer (grey line). (d) Schematics of the acetone absorption experiment. The shaded part represents the detector system, which in this case is included in the OSA. Figure 2b shows the optical frequency comb spectrum derived from the 700-μm-diameter resonator pumped with ~600 mW of laser power at λ =2.45 μm. We observed more than 100 modes spaced by 107 GHz (corresponding to a span of over 200 nm), which corresponds to the FSR of the resonator (FSR= c /(2 πRn eff )), where R is the cavity radius, c is the speed of light in vacuum and n eff is the effective refractive index. The resonator has high optical finesse F =1.2 × 10 5 . Optical sidebands can be generated once the parametric threshold is exceeded. The threshold for parametric oscillation can be estimated as the point where the Kerr nonlinearity-induced frequency shift Δ ω Kerr reaches half the cavity decay rate (the bi-stability point), that is, as Δ ω Kerr =( n 2 ωFP coupled )/(2 π nA eff )= κ /2, where n is the refractive index, n 2 the Kerr nonlinearity, P coupled the power coupled into the resonator, A eff the effective modal area, F the cavity finesse, κ the cavity decay rate and ω the optical angular frequency. The estimated threshold for sideband generation is P=4 mW, which matches the experimental observation. The power per generated comb line ranges from microwatts up to several milliwatts, significantly higher than the current state-of-the-art down-converted mid-infrared combs [9] , [10] . Figure 2: Mid-infrared optical frequency comb generation using a crystalline MgF 2 microresonator. ( a ) The experimental set-up consists of a CW mid- infrared OPO that serves as the pump laser. The pump laser is coupled via a tapered fibre to a crystalline MgF 2 microresonator. The generated frequency comb is detected using an optical spectrum analyser (OSA) with a cut-off wavelength of 2.5 μm (PD, photodetector). ( b ) Frequency comb spectrum recorded by the OSA around λ =2.45 μm with a line spacing of 107 GHz generated from pumping a 700-μm-diameter MgF 2 resonator (pump power 600 mW). The grey lines denote frequency components, which are expected to exist based on symmetry around the pump. Inset shows the spectrum taken with a Fourier transform spectrometer, which reveals the overall symmetry of the spectrum. ( c ) Proof-of-principle mid-infrared Kerr comb absorption spectroscopy experiment. The figure shows the transmittance of 0.5-mm-thick liquid acetone (single-pass) recorded as the relative intensities of the attenuated and unattenuated Kerr comb (shown in panel b ) line intensities (red dot) and independently by a Fourier transform spectrometer (grey line). ( d ) Schematics of the acetone absorption experiment. The shaded part represents the detector system, which in this case is included in the OSA. Full size image Prospects for spectroscopy Frequency combs have recently demonstrated potential for advances in molecular spectroscopy [35] , [36] . To demonstrate that the high power per comb line and the wide mode spacing is well suited for the recording of broadband vibrational spectra in the liquid or solid phase, we performed a proof-of-concept direct comb absorption spectroscopy [3] of 0.5 mm-thick layer of liquid acetone using the comb in Fig. 2b as light source and recording the transmission spectra with the OSA. Figure 2d shows the schematics of the comb spectroscopy. The result is shown in Fig. 2c and validated by an independent measurement of the same acetone sample employing a conventional white light source and a Fourier transform spectrometer (FTS). The discrepancy between the FTS and the comb measurements comes from the fact that the power in the resonator has not been stabilized in this work, and the comb line intensities fluctuate on a few seconds time scale required for data taking. Note that if a white light source is used for spectroscopy, a wavelength-calibrated detector system is required, whereas with a frequency comb source the calibration is contained in the known frequencies of the comb modes, and only a detector that can resolve the individual comb components is required. In future experiments employing a mid-infrared disperser and detector array, we expect microresonator-based combs to be suitable light sources for direct molecular fingerprinting [3] , which would vastly improve the acquisition time and sensitivity. Therefore, new opportunities for real-time spectroscopic investigation and optimization of chemical reactions may come into reach, including industrial real-time process control of, for example, pharmaceutical products. Phase noise characterization A key requirement of an optical frequency comb is low phase noise. Although parametric sidebands can already be generated in the weak anomalous dispersion region, it has been shown recently [30] that an anomalous dispersion parameter D 2 on the order of the cavity decay rate κ leads to intrinsically low-phase noise comb operation. The underlying physical picture is that the ratio κ / D 2 determines the position of the primary sidebands relative to the pump, and therefore the pathways of the comb formation process. For κ / D 2 >>1, the primary sidebands are far away from the pump and spectrally separated sub-combs form before merging, which results in multiple lines in a single optical cavity resonance. This leads to multiple beat notes (or more general phase noise) as well as amplitude noise [30] . In contrast, due to the strong anomalous dispersion of MgF 2 over the entire mid-infrared spectral range ( Fig. 1c ) and the high Q factors, a ratio of κ / D 2 ≈1 is attained in the mid-infrared. This results in primary sidebands close to the pump, such that intrinsically low-noise operation can be expected, as opposed to the telecom wavelength band where high-phase noise in the form of broad and multiple beat notes is frequently observed in crystalline, [30] silicon nitride [30] , [31] and fused quartz [25] resonators, and in toroids generating broadband spectra [19] . To investigate the noise [30] in the generated mid-infrared combs ( Fig. 3a ), one can either measure the repetition rate beat note, the heterodyne beat notes between a narrow-linewidth CW laser and the comb lines, or the amplitude noise. On the one hand, for a high-phase noise comb state, multiple or broad beat notes will be observed in the radio frequency domain, along with excess low-frequency amplitude noise [30] ; on the other hand, a low-phase noise comb state will have a single and narrow repetition rate or CW heterodyne beat note, and no additional amplitude noise. As ultra-fast mid-infrared detectors capable of detecting the repetition rate of tens of gigahertz frequencies are still in their development stage and not accessible for our experiment, we investigated in this work the phase noise of the mid-infrared Kerr combs by first, measuring the amplitude noise and second, by performing a CW heterodyne beat note measurement. 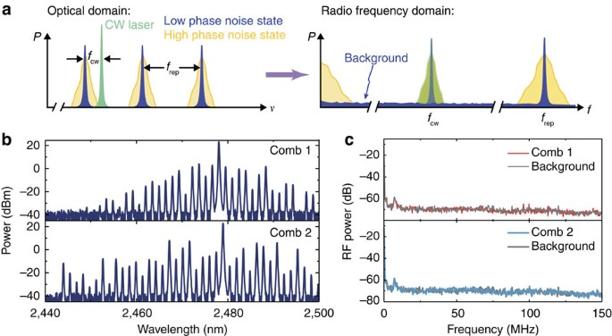Figure 3: Phase noise investigation of the mid-infrared frequency comb modes. (a) Illustration of how phase noise of the comb lines can be measured. A low-phase noise comb state (blue) will show a single, narrow repetition rate beat note and CW heterodyne beat note in the radio frequency domain, and no low-frequency amplitude noise; on the other hand, a high-phase noise state (yellow) will show multiple or broad beat notes in repetition rate or CW heterodyne measurement, and also excess low-frequency amplitude noise. Phase noise can thus be determined either by measuring the repetition rate beat note, the CW heterodyne beat note, or the amplitude noise of the comb. (b) Two comb spectra derived from a 1-mm-diameter resonator with a line spacing of 70 GHz. Panelcshows the amplitude noises of the two combs, which are the same as the detector noise background. It proves that the two combs have low phase noise. Figure 3b shows two comb spectra derived from a 1-mm-diameter resonator with a line spacing of 70 GHz. Their respective amplitude noise is shown in Fig. 3c along with the detector background noise. No additional noise is observed, indicating that the combs have low phase noise. The experimental set-up and results of the CW heterodyne beat note measurement are shown in Fig. 4 . 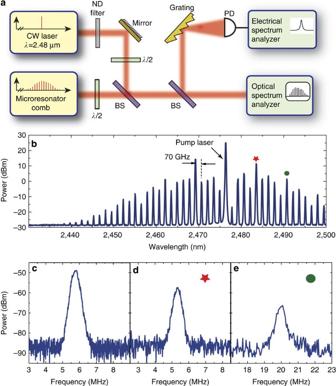Figure 4: Phase noise investigation of the mid-infrared frequency comb modes. (a) Experimental set-up of the CW laser beat note measurement. BS, beam splitter; PD, photodetector. (b) Frequency comb spectrum with a line spacing of 70 GHz used for the beat note measurement. Panelcshows the beat note between the CW laser and the pump, whereas panelsdandeshow the beat note between the CW laser and the comb modes (marked by the red star and the green dot inb, respectively). All beat notes have a full width at half maximum of ~300 kHz, corresponding to the resolution bandwidth used in the measurement. No other peaks are observed in the measurement with a larger frequency span. Beat notes between the CW laser and other comb modes show the same linewidth. Figure 4b shows the optical comb spectrum investigated, which was derived from the same resonator as in Fig. 3 . After measuring the beat of the CW laser with the narrow-linewidth pump ( Fig. 4c ), the beat notes between the CW laser and different comb modes were recorded ( Fig. 4d ). All beat notes exhibit the same linewidth corresponding to the employed resolution bandwidth of 300 kHz. Importantly, neither additional linewidth broadening of the comb modes relative to the pump nor multiple beat notes are observed in this measurement, showing that the comb lines exhibit a similar level of phase noise as the CW pump laser. We emphasize that the phase noise in the form of multiple or broad beat notes in Kerr frequency combs does not exhibit a dependence on frequency distance from the pump [30] . Figure 3: Phase noise investigation of the mid-infrared frequency comb modes. ( a ) Illustration of how phase noise of the comb lines can be measured. A low-phase noise comb state (blue) will show a single, narrow repetition rate beat note and CW heterodyne beat note in the radio frequency domain, and no low-frequency amplitude noise; on the other hand, a high-phase noise state (yellow) will show multiple or broad beat notes in repetition rate or CW heterodyne measurement, and also excess low-frequency amplitude noise. Phase noise can thus be determined either by measuring the repetition rate beat note, the CW heterodyne beat note, or the amplitude noise of the comb. ( b ) Two comb spectra derived from a 1-mm-diameter resonator with a line spacing of 70 GHz. Panel c shows the amplitude noises of the two combs, which are the same as the detector noise background. It proves that the two combs have low phase noise. Full size image Figure 4: Phase noise investigation of the mid-infrared frequency comb modes. ( a ) Experimental set-up of the CW laser beat note measurement. BS, beam splitter; PD, photodetector. ( b ) Frequency comb spectrum with a line spacing of 70 GHz used for the beat note measurement. Panel c shows the beat note between the CW laser and the pump, whereas panels d and e show the beat note between the CW laser and the comb modes (marked by the red star and the green dot in b , respectively). All beat notes have a full width at half maximum of ~300 kHz, corresponding to the resolution bandwidth used in the measurement. No other peaks are observed in the measurement with a larger frequency span. Beat notes between the CW laser and other comb modes show the same linewidth. Full size image As shown in the simulation in Fig. 1a , the magnitude of D 2 is monotonically increasing with wavelength above 1.55 μm in MgF 2 resonators (anomalous dispersion). Consequently, intrinsically low-phase noise Kerr combs can be expected across the entire mid-infrared region. This is in contrast to the telecom wavelength region around 1.5 μm, where we could not observe intrinsically low-noise states in the same resonators despite various pumping conditions, in agreement with the understanding of phase noise in ref. 30 . In the present work, the choice of pump wavelength of λ =2.45 μm originates from the current limitation of the available OSA and the coupling fibre's strongly increasing absorption beyond 2.5 μm. The first reason is not a limiting factor of the system itself and the fibre absorption may be circumvented by employing, for example, a coupling prism [37] or tapered chalcogenide fibres [38] instead. Pertaining to the advantages of crystalline microresonator-based mid-infrared frequency comb generators, it is noted that the native mode spacing in the range of 10–110 GHz is one unique feature. On the one hand, the comb repetition rate and carrier envelope offset frequencies are accessible with (suitably fast) photodetectors, electronics and digital signal processing; on the other hand, the comb modes may be individually accessed and even controlled. Indeed, a growing number of emerging applications require combs with large line spacing, such as astronomical spectrograph calibration, arbitrary optical waveform synthesis and spectroscopy [15] . Line-by-line pulse shaping of individual comb lines [39] may prove beneficial to coherent control of chemical reactions. Moreover the ability to dispersively separate the individual modes of the mid-infrared Kerr comb with a single grating onto a detector array enables direct fingerprinting of molecular absorption [3] . In summary, a crystalline microresonator-based optical frequency comb in the mid-infrared ‘molecular fingerprint’ region is demonstrated for the first time. This is also the first time that a Kerr comb is generated in the strongly anomalous dispersion region, which was previously considered unfavourable for Kerr comb generation. The high power per comb line and the potential to extend the comb to longer wavelengths makes it a promising candidate for spectroscopic applications. Moreover, the combination of crystalline microresonators with mid-infrared QCLs (which can generate high-CW output power at room temperature) could open the path to novel, simple and compact mid-infrared comb generators. Furthermore, the choice of the microresonator material is not limited to dielectric crystals. As many semiconductors such as silicon (Si), germanium (Ge) and indium phosphide (InP) also exhibit wide transparency windows in the mid-infrared and third-order nonlinearity (see Methods and Supplementary Table S2 ), a whole class of on-chip microresonator frequency combs for molecular spectrometers based on this approach is conceivable. Material choice The suitable platform for mid-infrared Kerr comb generation should possess the following properties simultaneously: wide transparency window in the mid-infrared; low loss for achieving high-Q cavity; Kerr nonlinearity n 2 ; anomalous GVD; the same signs of thermal coefficient of refractive index d n /d T and thermal expansion coefficient α . The last criterion comes from the thermal instability described in the Supplementary Note section, which has a key role for stable operation of Kerr combs. In Supplementary Table S1 , we list the dielectric crystal materials under consideration with their respective properties. All the materials have positive thermal expansion coefficients. As can be seen from Supplementary Table S1 , although most of the fluoride crystals have wide transparency window in the mid-infrared and anomalous GVD, they have negative d n /d T, which would induce thermal instability and render thermal self-locking inapplicable. Silicon nitride has a normal bulk GVD in the mid-infrared, and the current fabrication difficulty to grow Si 3 N 4 waveguides thicker than ~800 nm makes mode confinement and dispersion engineering very challenging. The two suitable materials for mid-infrared Kerr comb generation from the list would be MgF 2 and Al 2 O 3 . In this work, we choose MgF 2 because fluoride crystals (such as CaF 2 and MgF 2 ) have lower material absorption therefore could reach higher Q than Al 2 O 3 , especially for wavelength longer than 2 μm (ref. 40 ). In addition to dielectric crystals, many semiconductor materials also possess wide transparency windows in the mid-infrared and strong Kerr nonlinearity. The advantages of semiconductors are that they allow on-chip integration and are more versatile for waveguide dispersion engineering. Supplementary Table S2 lists several possible semiconductor materials for mid-infrared Kerr comb generation, including silicon (Si), germanium (Ge), aluminium nitride (AlN), gallium arsenide (GaAs) and indium phosphide (InP). The unwanted two-photon absorption is avoided once the photon energy is less than half the bandgap (for example, λ >2.2 μm for silicon), therefore the material loss is lower in the mid-infrared. While we do not find the experimental data on the bulk Kerr nonlinearity n 2 in the mid-infrared for AlN, GaAs and InP, it is expected to vary as E g −4 , where E g is the bandgap of the material [41] . Although Si and Ge have normal bulk material GVD in the mid-infrared, it is possible to create a spectral window of anomalous GVD by carefully designing the waveguide geometry. For example, for a Si ring resonator of radius 50 μm, width 900 nm and height 400 nm, it is expected that GVD would be anomalous between 2.0 and 3.2 μm. Set-up for microresonator-based mid-infrared frequency combs The employed pump laser is the idler beam of a high-power single-frequency, CW optical parametric oscillator (OPO) (Aculight Argos Model 2400). The pump of the OPO is a 15 W ytterbium-doped fibre-based source operating at 1064, nm, and the OPO is a four-mirror ring-resonant cavity using a temperature-controlled MgO-PPLN crystal as the nonlinear element. The idler beam is tuneable from 2.4 to 3.2 μm with up to 3 W output power, corresponding to a signal beam from 1.9 to 1.6 μm. The idler beam can be fine-tuned by piezoelectric tuning of the pump fibre laser. Both the idler and the signal beams have a specified linewidths of less than 1 MHz. The tapered-fibre waveguide is made of low-OH-fused silica fibre, which is single mode at 2.5 μm. The idler beam of the OPO was coupled into the tapered fibre by an AR-coated aspherical ZnSe lens. A coupling efficiency of more than 60% was obtained. The optical spectra of the combs were recorded by a Yokogawa long-range OSA. A second OPO, similar to the pump laser source, is used as the narrow-linewidth CW laser in the beat note measurement. The beat notes are recorded using an extended InGaAs detector with 100 MHz bandwidth. How to cite this article: Wang, C.Y. et al . Mid-infrared optical frequency combs at 2.5 μm based on crystalline microresonators. Nat. Commun . 4:1345 doi: 10.1038/ncomms2335 (2013).